Diastereomeric liquid crystal domains at the mesoscale In many technologies used to achieve separation of enantiomers, chiral selectors are designed to display differential affinity for the two enantiomers of a chiral compound. Such complexes are diastereomeric, differing in structure and free energy for the two enantiomers and enabling chiral discrimination. Here we present evidence for strong diastereomeric interaction effects at the mesoscale, manifested in chiral liquid crystal guest materials confined in a chiral, nanoporous network of semi-crystalline helical nanofilaments. The nanoporous host is itself an assembly of achiral, bent-core liquid crystal molecules that phase-separate into a conglomerate of 100 micron-scale, helical nanofilament domains that differ in structure only in the handedness of their homogeneous chirality. With the inclusion of a homochiral guest liquid crystal, these enantiomeric domains become diastereomeric, exhibiting unexpected and markedly different mesoscale structures and orientation transitions producing optical effects in which chirality has a dominant role. Since the first demonstration of the handedness of tartaric acid molecules by Pasteur [1] , resolution of enantiomers and dissymmetric induction in synthesis have been important from the perspectives of both science and technology [2] , [3] , [4] , [5] . In recent years, much effort has been expended on researching methods of fabricating nanoscale chiral surfaces, in many cases with the goal of improving enantioselectivity in asymmetric induction [6] , high-performance liquid chromatography [7] , [8] and high-sensitivity chirality detection [9] , [10] . Fabrication techniques include cleaving metal surfaces along low-symmetry planes [11] , adsorption of chiral molecules onto metal surfaces [12] , [13] , [14] , electrodeposition [15] , molecular imprinting [16] , [17] , [18] , glancing-angle deposition [19] and employment of metal-organic frameworks [20] . Liquid crystal (LC) systems have recently emerged as a promising class of materials exhibiting chiral interface effects, since they readily self-assemble into complex chiral structures in response to little more than appropriate sequences of changing temperature [21] . Liquid crystals exhibit a wide variety of chiral structures and responses, in both synthetically chiral systems and those where there is spontaneous reflection symmetry breaking, at lengths ranging from the molecular (in chiral bent-core phases, for example) to the macroscopic (as in the induction of chirality by micron-scale twist of the nematic director in a twisted cell geometry). During the last decade, spontaneous reflection symmetry breaking has been reported in several fluid LC phases of achiral bent-core molecules, with macroscopic, chiral conglomerate domains and a wide variety of novel structural phenomena involving the interplay of chiral, polar and liquid crystalline order observed in smectic phases of tilted molecules [22] , [23] , [24] , [25] , [26] , [27] , [28] , [29] . Among the novel phases exhibited by bent-core mesogens, the helical nanofilament (HNF) phase is one of the most fascinating and potentially useful. In this phase, also known as the B4, the bent-core molecules form well-defined smectic layers with in-plane hexatic order, and the combination of macroscopic polarization and molecular tilt makes the layers chiral ( Fig. 1a ). The layers are intrinsically unstable with respect to local saddle-splay distortion, a result of the internal stretch of the top and bottom halves of each smectic layer in nearly orthogonal directions ( Fig. 1b ), leading to the spontaneous formation of left- and right-handed helical nanofilaments ( Fig. 1c ) [30] , [31] . The preferred local radius of the saddle-splay ( R ∼ 25–30 nm) [30] is such that only saddle-splayed layers grow in upon cooling, so each filament becomes a chiral, twisted bundle of a few ( ∼ 8) smectic layers that is arbitrarily long (limited by the size of the cell, for example) but of finite diameter ( D ∼ 30 nm). Helical nanofilaments are unique among mesogenic structures with respect to their stability, reproducibility, and controllability. The HNF phase is one of the rare liquid crystal phases that preserves its nanoscale LC structure in a room temperature semi-crystalline state [32] . The nanofilaments can be aligned with self-assembled monolayers [33] , shearing [34] , topographic confinement [35] and controlled growth in a unidirectional director field [36] . Potential applications of HNFs utilize electric-field controlled optical activity in nano-segregated 5CB/HNF mixtures [37] , the enhanced optical activity of achiral, rod-like molecules nanosegregated in the HNF structure [38] or the self-assembled hydrophobic surfaces formed by toric focal conics and HNFs [39] . HNF networks can even form organogels that absorb large amounts of solvent at concentrations as low as 2 wt% (refs 40 , 41 ). 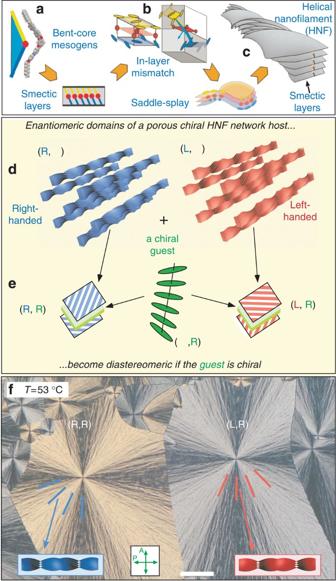Figure 1: Diastereomeric domains of a chiral guest mesogen infiltrated into left- and right-handed helical nanofilament networks of bent-core liquid crystal. (a–c) Hierarchical self-assembly of achiral bent-core mesogens into helical nanofilaments (diameter,D∼30 nm). (d–f) A typical HNF sample is a conglomerate of independently nucleated left- and right-handed domains many hundreds of microns across, each of which is a network of homochiral helical nanofilament bundles that acts as a mesoscale porous chiral host. (e) Owing to their chirality, the surface patterning on nanofilaments that locally face each other within a domain have different orientations, which causes the director field of an achiral nematic liquid crystal in the pores to twist along a line between these boundary orientations. When the guest nematic is chiral, however, it has spontaneous bulk twist with a well-defined handedness. Since the boundary conditions presented by the parallel nanofilaments in each of the chiral HNF domains are mirror images, the average director orientation of a chiral nematic relative to the long axis of the nanofilaments is different (diastereomeric) in the two domains, and they display macroscopically distinct optical properties. (f) Typical cell texture in a mixture of NOBOW with a chiral guest material (in this case, 50% 7O.5* by weight). The helical nanofilaments phase-separate from the isotropic melt at∼140 °C, nucleating at random sites in the cell surface and growing radially outwards to form homochiral, spherulitic domains with a local nematic-like texture of filaments (Supplementary Fig. 8). On average, we observe equal areas of left- and right-handed HNF domains in the cell. Scale bar, 100 μm. Unless otherwise specified, all cells used here were 3.2 μm thick. Schematic (a–c) is adapted from ref.30. Figure 1: Diastereomeric domains of a chiral guest mesogen infiltrated into left- and right-handed helical nanofilament networks of bent-core liquid crystal. ( a – c ) Hierarchical self-assembly of achiral bent-core mesogens into helical nanofilaments (diameter, D ∼ 30 nm). ( d – f ) A typical HNF sample is a conglomerate of independently nucleated left- and right-handed domains many hundreds of microns across, each of which is a network of homochiral helical nanofilament bundles that acts as a mesoscale porous chiral host. ( e ) Owing to their chirality, the surface patterning on nanofilaments that locally face each other within a domain have different orientations, which causes the director field of an achiral nematic liquid crystal in the pores to twist along a line between these boundary orientations. When the guest nematic is chiral, however, it has spontaneous bulk twist with a well-defined handedness. Since the boundary conditions presented by the parallel nanofilaments in each of the chiral HNF domains are mirror images, the average director orientation of a chiral nematic relative to the long axis of the nanofilaments is different (diastereomeric) in the two domains, and they display macroscopically distinct optical properties. ( f ) Typical cell texture in a mixture of NOBOW with a chiral guest material (in this case, 50% 7O.5* by weight). The helical nanofilaments phase-separate from the isotropic melt at ∼ 140 °C, nucleating at random sites in the cell surface and growing radially outwards to form homochiral, spherulitic domains with a local nematic-like texture of filaments ( Supplementary Fig. 8 ). On average, we observe equal areas of left- and right-handed HNF domains in the cell. Scale bar, 100 μm. Unless otherwise specified, all cells used here were 3.2 μm thick. Schematic ( a – c ) is adapted from ref. 30 . Full size image In binary mixtures of an HNF-forming bent-core host with many different mesogenic guest compounds, there is strong phase separation, with nanofilaments forming a nanoporous network and the guest material expelled from the HNFs to occupy the interstitial volumes between them [42] , [43] . In mixtures, the HNFs appear via a first-order phase transition, nucleating randomly at very dilute sites in a typical LC cell [44] . The initial nucleation event determines the handedness of the HNFs, which grow radially outwards from the nucleation site to form a spherulitic domain ( Fig. 1f ) that is completely homochiral, that is, every HNF grown in a given domain has the same handedness [45] , [46] . In each chiral domain, the guest material is nanoconfined to the pores of the HNF network, which has a large surface-area-to-volume ratio ( ∼ 100 m 2 cm −3 , comparable to aerogel) [40] , [41] . This geometry suggests that HNF networks might be useful in chiral separations or catalysis [47] , if the appropriate chemical distinctions can be exhibited by the HNF surface. In a typical preparation, there is a patchwork of left- and right-handed HNFs with roughly equal areas, distinguished generally by their optical rotation (OR) or birefringence colour, as in Fig. 1f . In a variety of applications, it would be desirable to engineer HNF networks that have the same chirality everywhere. Induction of globally homochiral, bent-core LC domains has been demonstrated by several methods, including controlled growth in a twisted director field [48] , using biomolecular adsorbates [49] and by mixing chiral dopants into the fluid B2 phase [50] . Homochiral samples can also be achieved by using structurally chiral bent-core mesogens [51] , [52] . To this end, we investigated in our experiments the properties of left- and right-HNF domains in binary mixtures of the prototypical achiral, HNF-forming bent-core mesogen NOBOW [53] mixed with a variety of chiral dopants. We found, with few exceptions, that the chosen chiral dopants, which include calamitic mesogens and cholesterol derivatives, had no observable effect on the proportion of left- and right-handed domains nucleated in the cell. These mixtures did, however, present an exciting new family of diastereomeric systems to explore, in which nanoporous networks with identical structure but opposite handedness host a chiral LC guest. The failure of the guests to cause chiral induction is likely a consequence of both the high temperature at which the HNFs form in the melt, with the transition into the HNF phase occurring when the guests are isotropic, and of the extremely low solubility of the guests in the HNFs, making the guest–HNF interaction weak at high temperature. As the temperature is reduced, however, the chiral guest acquires local and then macroscopic orientational and positional liquid crystal order within the confines of the left- or right-handed domains of the HNF network [54] , [55] . This guest–host coupling then becomes significantly enhanced, with the guest increasingly influenced by the difference between the diastereomeric domains as manifested in distinctive thermo-optical orientation effects. Nanoconfinement of guest molecules in NOBOW HNF networks Binary mixtures of NOBOW with a variety of guest materials (chiral, racemic and achiral) were prepared and studied. The chemical structures and phase sequences of neat NOBOW and the principally studied guest materials 8S5 (ref. 56 ) and 7O.5* (ref. 57 ) are shown in Fig. 2 , with the rest of the guests studied shown in Supplementary Figs 1–5 and Supplementary Table 1 . The notation ‘*’ indicates that a molecule and its phases (Iso*, N*, Sm* and so on) are chemically, and therefore structurally, chiral. The 8S5 and 70.5* mixtures with NOBOW, prepared with the guest material concentration, c , in the range 30 wt%< c <50 wt%, show similar global phase behaviour, indicated schematically in Supplementary Fig. 6 and described as follows. Above the HNF melting temperature, where the guests and NOBOW are isotropic as neat materials, the mixtures form a single, homogeneous isotropic (Iso) phase. On cooling, the NOBOW HNF phase appears first and strongly phase-separates from the isotropic solution. The HNF phase nucleates as internally homochiral, spherulitic domains from point nucleation sites that break achiral symmetry with a random distribution of handedness and grows upon cooling with smooth circular boundaries that advance until neighbouring domains meet ( Fig. 1f ). The HNFs are typically diluted by guest material and have a helical structure very similar to that of neat NOBOW, as confirmed by freeze-fracture transmission electron microscopy (FFTEM) observations ( Supplementary Fig. 7 ). Prior X-ray diffraction study [42] indicates the NOBOW/guest phase separation is nearly complete, with guest expelled from the interior and NOBOW similarly insoluble in the guest. FFTEM also shows that the HNFs are completely of a single handedness within each spherulitic domain. The principal optical characterization methods are measurement of optical rotation and birefringence, the former due to the HNF and/or guest chirality, and the latter driven by the local nematic-like orientational ordering of the HNFs in the host network, which is uniaxial about the mean HNF ( z ) axis, generating an average uniaxial birefringence Δn of the HNF/guest system ( Supplementary Fig. 8 ). This overall uniaxial symmetry will thus produce orientation distributions of the guest director f ( θ ) that are azimuthally symmetric about z ( Supplementary Fig. 9 ), with Δn ∝ 〈 P 2 (cos θ )〉 ≡ Q ( θ ), where θ is the polar orientation of a local dielectric tensor principal axis, e.g., the guest nematic director n ( r ), relative to z . The twist sense of the helical nanofilaments in the domains can be determined by combining OR measurements with FFTEM techniques (as explained in Supplementary Discussion 1 ) which show that, in the high temperature regime where the guests are isotropic, domains of right-handed (left-handed) HNFs rotate the polarization of visible light clockwise (counter-clockwise). In Figs 3 , 4 , 5 , and Supplementary Figs 10, 11, 12 and 16 , the notations (Iso), (N), (Sm) and so on indicate the phase of the (bulk) guest in the larger pores of the HNF network host. The phase transition temperatures of the guests in the HNF network are somewhat shifted (by < ∼ 10 °C) relative to their neat bulk values due to chemical instability of, and impurities in, the NOBOW host. 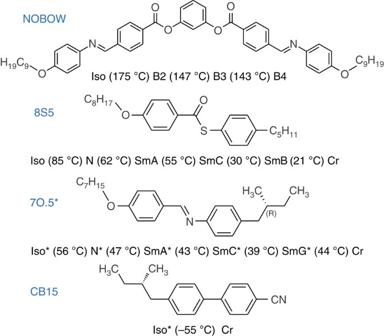Figure 2: Chemical structures and phase sequences of NOBOW (an achiral, bent-core LC), 8S5 (an achiral, rod-like LC), 7O.5* (a chiral, rod-like LC), and CB15 (a chiral dopant). Iso=isotropic; Iso*=chiral isotropic; N=nematic; N*=chiral nematic; Sm=smectic; Sm*=chiral smectic; Cr=crystal. Figure 2: Chemical structures and phase sequences of NOBOW (an achiral, bent-core LC), 8S5 (an achiral, rod-like LC), 7O.5* (a chiral, rod-like LC), and CB15 (a chiral dopant). Iso=isotropic; Iso*=chiral isotropic; N=nematic; N*=chiral nematic; Sm=smectic; Sm*=chiral smectic; Cr=crystal. 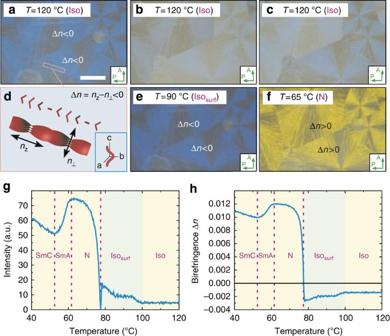Figure 3: Textures of HNF domains of an 8S5/NOBOW HNF network mixture. In ac=30% 8S5 (an achiral, rod-like LC)/NOBOW mixture, NOBOW phase-separates first on cooling from the isotropic blend, forming low-birefringence B4 domains (a) in which the helical nanofilaments grow radially outwards from a central nucleus and have very low birefringence (Δn=nz–n⊥∼0.001). The domains are chiral and cause optical rotation, revealed by decrossing the analyser (b,c). The 8S5 is still isotropic at this temperature (the guest phase is indicated in parentheses in all images). (d) Molecular and layer organization in a single HNF with refractive indicesnzandn⊥defined for the polarization directions indicated. The very low observed HNF birefringence is consistent with an estimate obtained by averaging values of the principal components of the optical dielectric tensor typical for bent-core mesogens,ɛa≈2.20,ɛb≈2.38 andɛc≈2.89 (ref.69), over the continuous reorientation around the filament axis (Supplementary Discussion 2). When the 8S5 transitions from Iso to N (e–f), the birefringence of both chiral domains becomes positive (Δn∼0.012), due to the additional contribution by the nanoconfined 8S5 nematic. However, thisΔnis much smaller than that which would be obtained if the nematic 8S5 were uniformly aligned (ne–no∼0.12, (Supplementary Fig. 10)). Such a reduction inΔnrequires a guest nematic director that is twisted in the pores, with a small net average orientation parallel to the local HNF axis. There is no observable difference between the left- and right-handed HNF domains between crossed polarizers at any temperature, indicating that they have the sameΔn. The scale bar in (a) is 100 μm. (g) Transmitted white light intensity through ac=30% 8S5/NOBOW cell between crossed polarizer and analyser. Incident light passes through a 30 μm diameter spot selected to be within a spherulite and to have the HNF axes making an average angle of 45° with respect to the polarizer axis. (h) Resulting measured birefringence,Δn. Moving to other positions in either L or R domains with polarizer and analyser crossed produces minor variations in the intensity curves due to the textures being slightly different. When 8S5, which is achiral, transitions from Iso to N, the birefringence of both chiral domains changes from negative to positive, giving a minimum in the transmitted intensity at around 78 °C. This change of sign shows that the growth of nematic order can produce ordering of sign different from that due to the surface ordering in the isotropic phase. The magnitude of the birefringence decreases as the 8S5 transitions from the nematic to the SmA phase, consistent with quasi-cylindrical guest smectic layers growing around the surfaces of the HNFs (as inFig. 7f). The bulk phase transitions of the 8S5 in the network are indicated as vertical dashed lines on the plots. Full size image Figure 3: Textures of HNF domains of an 8S5/NOBOW HNF network mixture. In a c= 30% 8S5 (an achiral, rod-like LC)/NOBOW mixture, NOBOW phase-separates first on cooling from the isotropic blend, forming low-birefringence B4 domains ( a ) in which the helical nanofilaments grow radially outwards from a central nucleus and have very low birefringence ( Δn=n z – n ⊥ ∼ 0.001). The domains are chiral and cause optical rotation, revealed by decrossing the analyser ( b , c ). The 8S5 is still isotropic at this temperature (the guest phase is indicated in parentheses in all images). ( d ) Molecular and layer organization in a single HNF with refractive indices n z and n ⊥ defined for the polarization directions indicated. The very low observed HNF birefringence is consistent with an estimate obtained by averaging values of the principal components of the optical dielectric tensor typical for bent-core mesogens, ɛ a ≈2.20, ɛ b ≈2.38 and ɛ c ≈2.89 (ref. 69 ), over the continuous reorientation around the filament axis ( Supplementary Discussion 2 ). When the 8S5 transitions from Iso to N ( e – f ), the birefringence of both chiral domains becomes positive ( Δn ∼ 0.012), due to the additional contribution by the nanoconfined 8S5 nematic. However, this Δn is much smaller than that which would be obtained if the nematic 8S5 were uniformly aligned ( n e –n o ∼ 0.12, ( Supplementary Fig. 10 )). Such a reduction in Δn requires a guest nematic director that is twisted in the pores, with a small net average orientation parallel to the local HNF axis. There is no observable difference between the left- and right-handed HNF domains between crossed polarizers at any temperature, indicating that they have the same Δn . The scale bar in ( a ) is 100 μm. ( g ) Transmitted white light intensity through a c= 30% 8S5/NOBOW cell between crossed polarizer and analyser. Incident light passes through a 30 μm diameter spot selected to be within a spherulite and to have the HNF axes making an average angle of 45° with respect to the polarizer axis. ( h ) Resulting measured birefringence, Δn . Moving to other positions in either L or R domains with polarizer and analyser crossed produces minor variations in the intensity curves due to the textures being slightly different. When 8S5, which is achiral, transitions from Iso to N, the birefringence of both chiral domains changes from negative to positive, giving a minimum in the transmitted intensity at around 78 °C. This change of sign shows that the growth of nematic order can produce ordering of sign different from that due to the surface ordering in the isotropic phase. The magnitude of the birefringence decreases as the 8S5 transitions from the nematic to the SmA phase, consistent with quasi-cylindrical guest smectic layers growing around the surfaces of the HNFs (as in Fig. 7f ). The bulk phase transitions of the 8S5 in the network are indicated as vertical dashed lines on the plots. 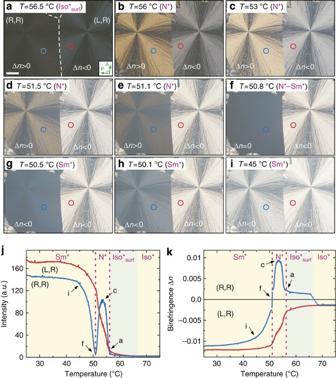Figure 4: Diastereomeric domains in a 7O.5*/NOBOW HNF network mixture. When the isotropic melt is cooled toT=70 °C in ac=50% 7O.5*(chiral, rod-like LC)/NOBOW mixture, the 7O.5* guest is still isotropic but NOBOW forms left- and right-handed HNF domains which have very low negative birefringence and appear dark under crossed polarizers. The scale bar is 100 μm. (a) At temperatures well above the bulk transition to the N*, the (L,R) and (R,R) domains develop birefringence of opposite sign at the Iso* to Iso*surftransition. (a–d) These signs are maintained at the Iso*surfto N* transition of 7O.5* where |Δn| grows substantially. (e–h) At the N* to Sm* transition, the birefringence in the (R,R) domain changes sign. At lower temperature, where the 7O.5* is smectic, all the domains have negative birefringence. (j) Transmitted light intensity,I, of the (R,R) and (L,R) domains as a function of temperature. The sampled regions (red and blue circles) have helical nanofilaments oriented approximately 45° from the crossed polarizer/analyser directions. (k) Spherulite birefringenceΔn(T) obtained fromΔn∝√I, with sign determination and calibration using a compensator. The bulk phase transitions of the 7O.5* in the network are indicated as vertical dashed lines on the plots. Full size image Figure 4: Diastereomeric domains in a 7O.5*/NOBOW HNF network mixture. When the isotropic melt is cooled to T= 70 °C in a c= 50% 7O.5*(chiral, rod-like LC)/NOBOW mixture, the 7O.5* guest is still isotropic but NOBOW forms left- and right-handed HNF domains which have very low negative birefringence and appear dark under crossed polarizers. The scale bar is 100 μm. ( a ) At temperatures well above the bulk transition to the N*, the (L,R) and (R,R) domains develop birefringence of opposite sign at the Iso* to Iso* surf transition. ( a – d ) These signs are maintained at the Iso* surf to N* transition of 7O.5* where | Δn | grows substantially. ( e – h ) At the N* to Sm* transition, the birefringence in the (R,R) domain changes sign. At lower temperature, where the 7O.5* is smectic, all the domains have negative birefringence. ( j ) Transmitted light intensity, I , of the (R,R) and (L,R) domains as a function of temperature. The sampled regions (red and blue circles) have helical nanofilaments oriented approximately 45° from the crossed polarizer/analyser directions. ( k ) Spherulite birefringence Δn ( T ) obtained from Δn ∝ √ I , with sign determination and calibration using a compensator. The bulk phase transitions of the 7O.5* in the network are indicated as vertical dashed lines on the plots. 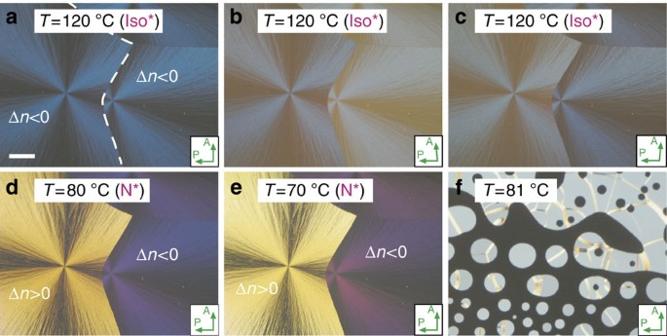Figure 5: Optical textures of a mixture of an achiral nematic mesogen and a chiral dopant with NOBOW. Ac=5% CB15/45% 8S5 in 50% NOBOW mixture is cooled from the isotropic until HNF domains appear. (a–c) At high temperature, where the guest material is Iso*, the chiral HNF domains of NOBOW exhibit very weak, negative birefringence. (d,e) Once the chiral guest mixture becomes nematic, the diastereomeric domains are optically distinct, as observed in the 7O.5*/NOBOW mixtures. (f) Typical cholesteric oily streak texture of thec=10% CB15/90% 8S5 mixture alone at the isotropic to chiral nematic transition. The scale bar in (a) is 100 μm. Note the hyperbolic boundaries between the domains, expected for adjacent domains growing from points at constant rates. Full size image Figure 5: Optical textures of a mixture of an achiral nematic mesogen and a chiral dopant with NOBOW. A c= 5% CB15/45% 8S5 in 50% NOBOW mixture is cooled from the isotropic until HNF domains appear. ( a – c ) At high temperature, where the guest material is Iso*, the chiral HNF domains of NOBOW exhibit very weak, negative birefringence. ( d , e ) Once the chiral guest mixture becomes nematic, the diastereomeric domains are optically distinct, as observed in the 7O.5*/NOBOW mixtures. ( f ) Typical cholesteric oily streak texture of the c= 10% CB15/90% 8S5 mixture alone at the isotropic to chiral nematic transition. The scale bar in ( a ) is 100 μm. Note the hyperbolic boundaries between the domains, expected for adjacent domains growing from points at constant rates. Full size image Even though the HNFs have local uniaxial ordering with preferred orientation along the radial growth direction ( Supplementary Fig. 8 ), and the NOBOW molecules are strongly optically anisotropic, the spherulitic domains of radial HNFs have only very low, negative, birefringence (| Δn | ∼ | n z – n ⊥ |< ∼ 0.001) when the HNFs have grown into a guest/NOBOW mixture that is isotropic (the usual case). This suggests that the low Δn is a result of orientational averaging of the local biaxial optical dielectric tensor director field within each HNF ( Fig. 3d and Supplementary Discussion 2 ), and that around the as-formed HNFs there is little orientation of the confined guest at high T , even at the guest/HNF interfaces. The general structural behaviour of achiral 8S5 and chiral 7O.5* as guests in NOBOW HNF networks is as follows. 8S5 (achiral)/NOBOW mixtures Because 8S5 is achiral, the left- and right-handed HNF domains in this mixture are enantiomeric, and thus their textures exhibit mirror-symmetric optical rotation as revealed by decrossing of the polarizers ( Fig. 3b,c ), and are therefore indistinguishable on average when viewed between crossed polarizers. As noted above, Δn of the 8S5/HNF system is very low when 8S5 is in the Iso phase ( Fig. 3a,h ). However, previous differential scanning calorimetry (DSC) and nuclear magnetic resonance (NMR) study [54] , [55] shows that the 8S5/NOBOW and 8CB/NOBOW mixtures exhibit a nematic surface alignment by which the guest forms a several nanometer-thick oriented layer on the HNF surface at lower temperatures in the guest isotropic phase (at T ∼ 90 °C for 8S5). This surface alignment is referred to as the isotropic surface-aligned state (Iso surf ) and is detectable in 8S5/NOBOW Δn data ( Fig. 3h ), giving a contribution Δn ∼ −0.001 starting just above the 8S5 Iso—N transition. As the 8S5/NOBOW mixture is further cooled a distinct transition in Δn is observed at T =77 °C ( Fig. 3h ) where nematic ordering appears in the confined guest ( Fig. 3e,f ) and the birefringence of domains of both handedness changes sign, becoming positive and growing substantially in magnitude ( Δn ∼ 0.012), but still remaining much smaller than that of aligned monodomain nematic 8S5 ( Δn ∼ 0.12, see Supplementary Fig. 10 ). Δn decreases in magnitude at the N—smectic A transition as a result of quasi-cylindrical 8S5 smectic layers growing around the surface of the HNFs (discussed below). 7O.5* (chiral)/NOBOW mixtures With the chiral guest material 7O.5*, on the other hand, the domains of opposite HNF handedness are structurally diastereomeric ((R,R): right-handed HNFs with right-handed 7O.5* nematic twist sense; (L,R): left-handed HNFs with right-handed 7O.5* nematic twist sense), and generally exhibit non-mirror symmetric chiral optical behaviour, such as that shown in Figs 1f and 4 , and Supplementary Figs 11 and 12 , for a c= 50% 7O.5*/NOBOW mixture, with 7O.5* in the chiral nematic (N*) phase. When the mixture is cooled from the isotropic melt, NOBOW domains nucleate at T= 140 °C while the 7O.5* is still isotropic (Iso*). Both left- and right-handed domains are observed with equal probability ( Fig. 1f ), a result of the essentially complete phase separation of the mixture that reduces the possibility of significant chiral induction by the chiral guest molecules. Upon cooling, isotropic 7O.5* also exhibits an Iso* to Iso* surf transition at which an oriented LC layer on the HNF surfaces appears [54] , [55] at T ≈ 70 °C, as indicated optically by the sign change of Δn of the (R,R) domain and by DSC ( Supplementary Fig. 13 ). The Iso* surf state for T <70 °C is also marked optically by an increasingly positive birefringence of the (R,R) domains ( Fig. 4j,k , Supplementary Fig. 11 ), and an increasingly negative birefringence of the (L,R) domains, a clear manifestation of the diastereomeric nature of the 7O.5* nanoconfinement, at the earliest stages of its ordering. Upon further cooling, the 7O.5* undergoes the Iso* surf −N* phase transition within the HNF network, also indicated by DSC, and by a strong increase in | Δn |, with Δn remaining positive in the (R,R) domains and negative in the (L,R) domains ( Fig. 4b–e , Supplementary Figs 11 and 12 ). As the N*—smectic A* (Sm*) transition is approached, the Δn of the (R,R) domains begins to significantly decrease, crossing zero to produce a striking extinction at T =50.8 °C, homogeneously within each (R,R) domain, and simultaneously throughout all of the (R,R) domains of the sample ( Fig. 4f ). This reversal of Δn is due to quasi-cylindrical 7O.5* smectic layers growing around and enveloping the surface of the HNFs, observable using FFTEM (discussed below). Thus, for T <50.8 °C the Δn of the (R,R) domains becomes negative, again with the same sign as that of the (L,R) domains ( Fig. 4g–i ). This results in the (R,R) domains having a range of T with positive Δn , while the (L,R) domains have negative birefringence at all T , a mesoscopic manifestation of their diastereomeric nature. CB15 (chiral dopant)/8S5 (achiral)/NOBOW mixtures Adding a chiral dopant to the 8S5/NOBOW system induces striking diastereomeric behaviour even at quite low dopant concentration. For example, in Fig. 5 , a c =5% CB15/45% 8S5/50% NOBOW mixture is cooled from the isotropic until HNF domains appear. At high temperature, where the guest material is Iso*, the chiral HNF domains of NOBOW exhibit very weak, negative birefringence and opposite OR, as for achiral 8S5 ( Fig. 5a–c ). However, the diastereomeric nature of the domains becomes optically very evident in the N* phase, with only one handedness of the HNF domains changing sign of Δn at the transition (as was also observed in the 7O.5*/NOBOW mixtures). Optical, LC ordering and surface anchoring characteristics This study focuses on HNF/guest systems where the bulk guests have an isotropic—nematic—smectic phase sequence, as summarized in Supplementary Table 1 . These systems generally exhibit three transitions between four distinct HNF-confined states of the guest as T is lowered: isotropic (Iso or Iso*)—no measurable guest alignment at the temperatures immediately below that of the HNF network formation; isotropic surface aligned (Iso surf or Iso* surf )—a transition in the Iso phase of the guest to surface-induced alignment of the guest on the HNFs, with the guest contributing Δn guest , of magnitude | Δn guest | ∼ 0.001 to the birefringence. This Δn guest can be of either sign, depending on the guest and/or the HNF handedness nematic (N or N*)—the Iso−N transition of the bulk guest, marked by a sharp increase in | Δn guest |, up to the | Δn guest | ∼ 0.01 range. For achiral guests the sign of Δn may or may not change at the Iso-N transition (the same in both L and R HNF domains of course), whereas for chiral guests at the Iso*-N* transition, Δn guest becomes distinctly different in the two domains with either the (L,R) or (R,R) changing sign at the transition, depending on the guest; smectic (Sm or Sm*)—the N-Sm transition of the bulk guest where the smectic contribution to Δn guest is increasingly negative with decreasing T and as large in magnitude as | Δn guest | ∼ 0.02. However, the nanoconfined guest/NOBOW HNF network systems consistently have an overall birefringence that is much smaller than that of the strongly birefringent, oriented bulk phases of the guest and/or NOBOW, in the range of 1 to 10% of the latter [55] , [56] . Such ratios require subwavelength orientational averaging of the guest LC optical anisotropy in which a significant fraction of the anisotropic molecular components have their high polarizability axes making a substantial angle θ with the HNF. This is the case in the fixed helical internal structure of the HNFs, where averaging of the bent-core molecular orientation gives rise to the low Δn HNF ( Supplementary Discussion 2 ). In an analogous manner, the low or negative Δn of the guest LC phases must arise from similarly large θ values, in the form of the heliconical director distribution about each HNF shown in Fig. 6c and discussed in Supplementary Fig. 9 . Such director distributions require strong anchoring on the HNF surfaces to be maintained, that is, with a surface penetration length, l , (ref. 58 ) much smaller than the HNF diameter, D ∼ 30 nm. Otherwise, if the anchoring were weak ( l > D ), the HNFs would act as a homogeneous uniaxial orienting force aligning the guest nematic with θ ∼ 0°, parallel to the HNFs and giving essentially its bulk Δn like a nematic monodomain stabilized by a dilute anisotropic polymer network [59] . Equations 1 and 2 in Supplementary Discussion 2 provide a means of estimating the average birefringence change produced by regions within the network of aligned guest, calculating the contribution to Δn due to a birefringent guest layer of uniform thickness w on the HNF surfaces. Taking the bulk nematic guest optical dielectric anisotropy to be Δɛ N =0.6 and the average guest refractive index to be n b =1.6, we find the estimated guest contribution to Δn to be Δn guest ∼ 0.012 × w (nm) × 〈 P 2 (cos θ )〉, or Δn guest ∼ 0.012*〈 P 2 (cos θ )〉 for a surface film that is about a single molecular monolayer in thickness ( w ∼ 1 nm). 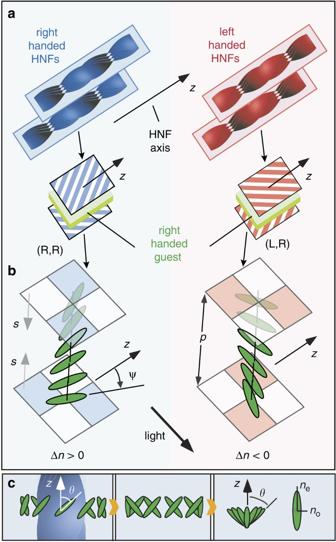Figure 6: Model of molecular organization in large-pore 7O.5*/HNF network domains. (a,b) The HNF network is approximated as an array of sheets of HNFs separated by pore dimensionp. For the case of 7O.5*, the pore is filled by guest mesogens preferring a right-handed twist of directorn(r), with a pitch∼300 nm. The structure adopted byn(r) in the pore is determined by the strong nanoheterogeneous anchoring on the HNF surfaces, which reflects the HNF chirality, as in (c), but, in the larger pores, anneals to a soft, chiral anchoring potential of the formW(ψ)=Wosin(2ψ) on each surface. The functional dependence ofW(ψ) onψis represented by 2 × 2 checkerboards, where quadrants inψwith minima (maxima) inψare shaded (unshaded). MinimizingW(ψ) by orientingn(r) near the HNF surfaces in the shaded quadrants leads to a macroscopic, optical manifestation of the diastereomeric nature of the system, givingΔn>0 andΔn<0 respectively in the (R,R) and (L,R) cases. (c) The overall guest/HNFΔnis a uniaxial spatial average of the distributionf(θ) of tilts of the localn(r) from the mean HNF axis,z. Figure 6: Model of molecular organization in large-pore 7O.5*/HNF network domains. ( a , b ) The HNF network is approximated as an array of sheets of HNFs separated by pore dimension p . For the case of 7O.5*, the pore is filled by guest mesogens preferring a right-handed twist of director n ( r ), with a pitch ∼ 300 nm. The structure adopted by n ( r ) in the pore is determined by the strong nanoheterogeneous anchoring on the HNF surfaces, which reflects the HNF chirality, as in ( c ), but, in the larger pores, anneals to a soft, chiral anchoring potential of the form W ( ψ )= W o sin(2 ψ ) on each surface. The functional dependence of W ( ψ ) on ψ is represented by 2 × 2 checkerboards, where quadrants in ψ with minima (maxima) in ψ are shaded (unshaded). Minimizing W ( ψ ) by orienting n ( r ) near the HNF surfaces in the shaded quadrants leads to a macroscopic, optical manifestation of the diastereomeric nature of the system, giving Δn >0 and Δn <0 respectively in the (R,R) and (L,R) cases. ( c ) The overall guest/HNF Δn is a uniaxial spatial average of the distribution f ( θ ) of tilts of the local n ( r ) from the mean HNF axis, z . Full size image Isotropic surface aligned . Nanometre-thick films of aligned nematic on solid surfaces in contact with the isotropic phase of a nematic LC are well known [60] , [61] , [62] . Applying the estimate of w ∼ 1 nm to the isotropic surface-aligned state of 7O.5*, where the contribution of the guest molecules to Δn in the (R,R) and (R,L) domains changes by, respectively, Δn guest(R,R) ∼ +0.003 and Δn guest(L,R) ∼ −0.001, that is, it is both small and diastereomeric, shows that either 〈 P 2 (cos θ )〉 must be small (〈 P 2 (cos θ )〉 ∼ 0.1), due to orientation on the HNFs near θ m , or that there is low nematic-like order of the local HNF axes, or that the average HNF surface-oriented film thickness must be substantially less than w =1 nm, that is, that there can be only partial, perhaps intermittent, coverage of the HNF surfaces. In any case, the manifestation of the diastereomeric nature of the (R,R) and (L,R) domains in so little ordered guest indicates that the earliest stages of ordering of the guest must take place at the HNF surfaces, where the HNF chirality can play a role. This, in turn, suggests the importance in the early stages of guest material confined in the smallest inter-HNF gaps (ranging in size from contact to a few nm). Nematic Turning to the nematic state of 7O.5*, assuming that the guest volume is now filled ( f =0.5), and again taking Δɛ N =0.6 and n b =1.6, we find Δn guest ∼ 0.1 × 〈 P 2 (cos θ )〉 from equation 1 of Supplementary Discussion 2 . If 〈 P 2 (cos θ )〉 ∼ 1, this is also much larger than the measured birefringence, | Δn guest | ∼ 0.01. In the nematic ordering of the guest/HNF systems, DSC data, such as Supplementary Fig. 13 , indicate that guest nematic order extends over >75% of the available volume. As the nematic order is filling the guest volume, the distribution of pore sizes P ( p ) in the HNF network, ranging from HNFs in contact to those spaced by hundreds of nanometres [40] , must be taken into account. Filamentary networks typically have lognormal pore size distributions with extended tails for larger pore sizes [63] , visible up to the micron scale in the FFTEM of mixtures [42] . Thus, if the HNF-confined 7O.5* has typical nematic local ordering then its director n ( r ) must be substantially disordered. Evidence for the nature of this disorder is provided by measurement of the electro-optic response of an 8CB/NOBOW guest/HNF system, as detailed in Supplementary Discussion 3 and Supplementary Fig. 14 . Here we find that an applied AC electric field that is large enough to orient the guest only in the largest pores of the HNF network (dimension p > ∼ 70 nm) reduces Δn of the spherulitic domains to the Δn ∼ 0.001 level, comparable to that of the isotropic surface-aligned state. Thus, the nematic director is rendered nearly isotropic by the HNF nanoconfinement in the smaller pores ( p < ∼ 70 nm), where the guest attains a fixed director field conforming to the HNF surface orientation preferences. Strong anchoring on the HNF surfaces combines with their mixed homeotropic and planar aligning faces and the overall orientational averaging due to HNF twist to render the small pores permanently nearly isotropic ( Supplementary Discussion 4 ). By contrast, the guest director n ( r ) in the larger pores, while also bounded by surfaces with strong anchoring, has enough space to reorder and anneal according to the dictates of its elasticity, inherent chirality and chiral HNF anchoring. Thus, we find that the contrasting (L,R) and (R,R) optical behaviour in the nematic state is a manifestation of the differing molecular organizations of the nematic 7O.5* director n ( r ) in the largest pores of the left- and right-handed HNF networks, respectively. In both of these domains the guest molecules adopt the right-handed twist direction preferred in the bulk N* phase ( Supplementary Fig. 15 ), subject to constraints of the twisted boundary orientations imposed by the nearest HNFs, which differ in the (R,R) and (L,R) domains ( Fig. 1d ). The behaviour of n ( r ) in the larger pores can be described by the model sketched in Fig. 1d , where the guest is taken to be in a planar slab between walls of HNFs oriented according to the (L,R) or (R,R) chirality, red or blue, respectively. The HNF walls act on the director field of the guest as strongly anchoring, nanotextured sheets, with n ( r ) disordered on the nanoscale near the HNF sheets but annealing to order out to larger length scales with increasing distance from the HNFs, a scale comparable to the pore dimension in the middle of a pore. This results in an effective orientational anchoring that is much weaker than that on the HNF surface, in the same way that solid substrates having random orientations patterned on the nanoscale produce nearly-degenerate azimuthal alignment of a contacting bulk nematic [64] , [65] , [66] , [67] . To describe the surface anchoring of 7O.5* on the HNFs we first explore having a preferred orientation of n ( r ) along the layer edge directions on the HNF surfaces ( Figs 1c and 7 , Supplementary Fig. 8 ), which locally make a substantial angle (>30°) with the HNF axis. The resulting remnant surface interaction reflecting the surface patterning and thus the chirality of the HNFs is described by a chiral Rapini-Papoular energy on each HNF sheet of the form W ( ψ )= W 0 sin(2 ψ ), the lowest order chiral term in a harmonic expansion of W ( ψ ). Here ψ is the angle defined at each pore surface between n ( r ) and z such that n ( r ) at the surface is given by n ( ψ )= z cos ψ +( z × s )sin ψ , where s is the surface normal pointing into the pore ( Fig. 6b ). In the (R,R) case, on the top surface of the pore in Fig. 6 , W 0 >0, and on the bottom surface, W 0 <0, with the sign of W 0 reversed in the (L,R) case. The 2 × 2 checkerboards in Fig. 6b sketch W ( ψ ) at each of the pore/HNF interfaces in the (L,R) and (R,R) pores, where in each case the shaded squares in the checkerboard indicate quadrants in ψ where W ( ψ )<0 (the preferred orientations of n ( ψ ) at the surface), and the white squares where W ( ψ )>0 (the non-preferred orientations of n ( ψ ) at the surface). As these anchoring potentials are very weak they do not substantially distort the right-handed bulk helix of 7O.5*. Rather, the helix maintains its pitch but simply reorients as a whole as a means of reducing its surface energy, a condition that is generally satisfied if n ( ψ ) at both surfaces of a pore (both ends of the guest helix) can simultaneously reorient into a shaded area. The resulting energy-minimizing n ( r ) fields achieving this condition for (L,R) and (R,R) pores of size p ∼ P guest /6 are sketched in Fig. 6b for nematic 7O.5*, along with the sign of the contribution of these orientation fields to Δn . 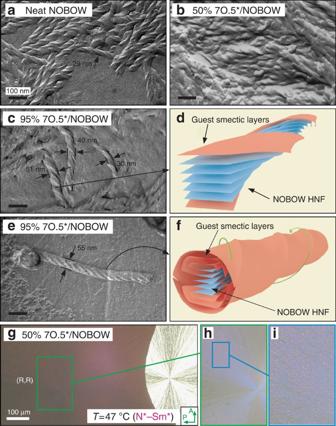Figure 7: Guest ordering into the smectic phase in an HNF network. (a) FFTEM image of neat NOBOW HNFs, in which the typical HNF diameter is∼30 nm and layer edges are clearly visible. (b) FFTEM image ofc=50% 7O.5*/NOBOW mixture atT=45 °C (where 7O.5* is in the smectic phase), showing a dense array of smooth HNFs with no visible layer edges. (c,e) HNFs are much more dilute in ac=95% 7O.5*/NOBOW mixture, enabling visualization of smectic growth around single HNFs, conformally on the surface of the HNFs in the case of 7O.5*. (c–f) Continuous sheath around the HNFs, hiding the layer edges but not the underlying helical structure. The scale bars in (a–c,e) are 100 nm. (g–i) Submicron scale speckles at the N*–Sm* transition of 7O.5* in ac=50% 7O.5*/NOBOW mixture reveal N* and Sm* subdomains coexisting over the same narrow range ofTeverywhere in the spherulite. This suggests a statistical distribution of local transition temperatures related to statistical fluctuations in the network. Figure 7: Guest ordering into the smectic phase in an HNF network. ( a ) FFTEM image of neat NOBOW HNFs, in which the typical HNF diameter is ∼ 30 nm and layer edges are clearly visible. ( b ) FFTEM image of c= 50% 7O.5*/NOBOW mixture at T= 45 °C (where 7O.5* is in the smectic phase), showing a dense array of smooth HNFs with no visible layer edges. ( c , e ) HNFs are much more dilute in a c= 95% 7O.5*/NOBOW mixture, enabling visualization of smectic growth around single HNFs, conformally on the surface of the HNFs in the case of 7O.5*. ( c – f ) Continuous sheath around the HNFs, hiding the layer edges but not the underlying helical structure. The scale bars in ( a – c , e ) are 100 nm. ( g – i ) Submicron scale speckles at the N*–Sm* transition of 7O.5* in a c= 50% 7O.5*/NOBOW mixture reveal N* and Sm* subdomains coexisting over the same narrow range of T everywhere in the spherulite. This suggests a statistical distribution of local transition temperatures related to statistical fluctuations in the network. Full size image In the case of (L,R) or (R,R) domains with 7O.5*, the polar orientation of n ( r ) is, respectively, larger or smaller than the magic angle θ m in Supplementary Fig. 9 , giving, respectively, Δn <0 or Δn >0. In larger pores with p > P guest /4, n ( r ) will exhibit an integral number of ( P guest /4)-thick slabs in each of which there is a π/4 rotation of n ( r ) and averaging over a similar range of θ , which contribute weakly to Δn , plus some remnant length. The surface energy and Δn calculations are then applied only to the remnant tail and the contribution of the pore to the average Δn is correspondingly reduced. In the same way, the larger pores contribute to the enhanced OR in 5CB/NOBOW systems observed by Otani et al . [38] Smectic . At lower temperatures the nematic to smectic transition of the nanoconfined guests takes place, producing changes in both their bulk nematic and surface alignment behaviour, including a substantial increase in the pitch for chiral nematic guests in the larger pores. Smectic layers begin to form in the pores, and in 7O.5* Δn in the (R,R) domains eventually changes sign so that the birefringence in both domains is again negative, implying that in the smectic guest material the high-index axis makes a substantial angle θ with the nanofilament axis ( Fig. 6c , Supplementary Fig. 9 ). To further investigate this smectic ordering, we performed FFTEM studies of calamitic guest/NOBOW mixtures with the guest in the smectic phase. Molecular order near the HNFs is more clearly observed in mixtures where the NOBOW is very dilute. Thus, with c= 95% 7O.5*/NOBOW the HNFs come out of the melt at T= 78 °C, well above the bulk isotropic to chiral nematic phase transition of 7O.5* and are well-separated, enabling observation of the morphology of the guest smectic material near single HNFs. The FFTEM images ( Fig. 7c,e ) reveal filament structures with a range of diameters larger than the bare HNFs (30 nm< D <55 nm) and very few exposed layer edges, giving an appearance consistent with conformal growth of guest smectic layers on the layer surfaces of the HNFs ( Fig. 7c,d ), with the guest smectic tending to enhance the characteristic screw-like appearance of the HNFs. Such a cylindrical SmA layer corresponds to the conical distribution of molecular orientations of Supplementary Fig. 9 with θ =90°, clearly contributing negative birefringence to Δn in both the (R,R) and (L,R) domains. We also observe thicker, smoother-coated HNFs that are more cylindrical but have a rope-like surface topography reminiscent of the underlying helical structure ( Fig. 7e,f ), confirming that the 7O.5* smectic layers coat the HNF surfaces. At higher NOBOW concentrations ( c= 50% 7O.5*/NOBOW at T= 45 °C in Fig. 7b ), the HNFs also show very few of the layer edges seen in neat NOBOW, implying that the nanofilaments are coated by the smectic layers of the guest material over a broad concentration range. The extinguishing state near T =50.8 °C is imaged at long exposure times in Fig. 7g–i and Supplementary Fig. 12 , showing that it is a speckle-like mosaic of micron-scale red ( Δn ∼ 0.002) and blue ( Δn ∼ −0.002) spots within the (R,R) domains. These spots can be taken as evidence for there being a range δT z of local zero-crossing temperatures for Δn ( T ). From the minimum birefringence of the spots of | Δn | ∼ 0.002, and the slope of Δn ( T ) near the crossing from Fig. 4k of d Δn ( T )/d T ∼ 0.004/°C we estimate δT z as δT z ∼ 0.002/(d Δn ( T )/d T ) ∼ 0.5 °C, a quite small range, indicating a quite homogeneous intrapore structure and environment throughout the sample, even at the centres of the spherulitic domains. The striking phase behaviour of enantiomeric or diastereomeric guest/HNF systems has been explored in many mixtures of the HNF-forming bent-core molecule NOBOW with, respectively, nonchiral (achiral, racemic) or chiral guest materials. As a function of temperature, these systems generally exhibit distinguishable isotropic, isotropic surface aligned, nematic and smectic HNF-confined guest states, as manifest optically by the overall birefringence and optical rotation, for example. In a given sample these states are obtained throughout the HNF network and the transitions between them take place homogeneously at distinct transition temperatures. Summarizing the nematic state in the guest/HNF systems, if the guest were in a weakly orienting network Δn would be uniaxial with Δn ∼ Δn guest /2, reflecting uniform uniaxial alignment of the guest. Measured Δn are ∼ 10% of this value, a result that can be achieved only with strong anchoring on the HNFs, enabling the combined disordering effects of the orientation variations in the local HNF axes ( Fig. 7b and Supplementary Fig. 8 ), HNF surface alignment-induced cancellation of Δn in the smaller pores ( Supplementary Fig. 14 ), and the fractional filling of, and orientational averaging in, the larger pores ( Fig. 6b ). The homogeneous mesoscopic diastereomeric behaviour implied by the ultra-low network birefringence at temperatures where the guest state changes is a result of the mesoscopic homogeneity of the HNF network and the nematic elastic annealing of the HNF anchoring distortions away from the HNFs in the larger pores. Apart from the isotropic phase, the particular structures of the guest in these various states and the changes observed at the transitions are not universal but, as indicated by Δn , rather appear to depend on the details of the orientational interactions of the guest at the HNF/guest interfaces. Thus, Δn may or may not be the same in the Iso guest and N states, the nematic diastereomeric domains may or may not have opposite sign of Δn , and even the smectic layering can induce positive rather than the negative Δn given by homeotropic orientation in the HNF as discussed above, for example, in cholesterol derivatives such as cholesteryl nonanoate ( Supplementary Figs 16 and 17 ). Such features of the polymorphism of the guest/NOBOW mixtures investigated are summarized in Supplementary Table 1 . Limited experimentation has also been carried out on guest/bent-core mixtures using other HNF-forming materials. These bent-core systems, such as W513 (ref. 68 ), exhibit similar multi-state phenomenology, typified by the 7O.5*/W513 mixture shown in Supplementary Fig. 18 . For all mixtures in which the guest material has a chiral nematic phase, the diastereomeric domains are easily distinguished in the microscope. The experiments reported here detail the structural guest/host behaviour of a class of chiral nanoporous host networks formed by self-assembly and spontaneous symmetry breaking in systems of bent-core liquid crystals. The resulting characterization of guest structure constitutes a general and necessary approach to the development of an understanding of chirality at the nanoscale and its mesoscopic manifestations, particularly if liquid crystal ordering is present or exploited, as a path towards applications in chiral separations and asymmetric synthesis. Optical observations were made using a Nikon Eclipse E400 POL microscope with polarizer and analyser equipped with an Olympus Camedia C-5050 Zoom digital camera. Birefringence was measured either using a Zeiss rotary compensator with quartz plates, or by converting intensity measurement as in Figs 3g and 4j to birefringence using the compensator as calibration. Optical rotation (OR) was measured by decrossing the polarizer and analyser. The liquid crystal mixtures were filled into Instec 3.2-μm commercial cells by capillary action at high temperature in the isotropic phase. Temperature was controlled using an Instec STC200D temperature controller. The samples were typically cooled slowly from the isotropic phase (at ∼ −2 °C min −1 ) to avoid any hysteresis effects. Freeze-fracture transmission electron microscopy experiments were carried out by sandwiching the sample between 2 mm by 3 mm glass planchettes and cooling from the isotropic phase to the desired phase while observing the sample in the microscope. The sample was then rapidly quenched to T <−180 °C by immersion in liquid propane, and fractured under high vacuum at −140 °C. It was subsequently coated with 2 nm of platinum deposited at a 45° angle, followed by ∼ 25 nm of carbon deposited at a 90° angle to increase the mechanical rigidity of the replica. After dissolving the liquid crystal, the Pt–C replica was placed on a copper grid and observed in a Philips CM10 100 keV TEM, where the topography of the fracture plane could be observed. Images were taken with a TEM-mounted 1 K × 1 K Gatan Bioscan digital camera. The surfaces facing the platinum shadowing direction accumulate more platinum and therefore produce darker shadows in the TEM images, revealing height variations in the topography. Differential scanning calorimetry measurements were carried out using a Mettler Toledo DSC823e/700. Materials CB15 (4-(2-methylbutyl)-4′-cyanobiphenyl) was purchased from Alfa Aesar. NOBOW (4-[[(E)-[4-(nonyloxy)phenyl]imino]methyl]-1,3-phenylene benzoate) was synthesized following the Matsunaga method, with a slight modification of the condensation step using N , N ′-carbonyldiimidazole (CDI) instead of dicyclohexyl carbodiimide (DCC) in the final esterification [53] . 8barS5 (8S5) (4-(Octlyoxy)benzenecarbothioic acid S-(4-pentylphenyl) ester) was synthesized according to the method in ref. 56 . 7O.5* (Benzenamine, N-[[4-(heptyloxy)phenyl]methylene]-4-(2-methylbuytl)-,(R)-) was synthesized according to the method in ref. 57 . How to cite this article: Chen, D. et al . Diastereomeric liquid crystal domains at the mesoscale. Nat. Commun . 6:7763 doi: 10.1038/ncomms8763 (2015).